Coupled local translation and degradation regulate growth cone collapse Local translation mediates axonal responses to Semaphorin3A (Sema3A) and other guidance cues. However, only a subset of the axonal proteome is locally synthesized, whereas most proteins are trafficked from the soma. The reason why only specific proteins are locally synthesized is unknown. Here we show that local protein synthesis and degradation are linked events in growth cones. We find that growth cones exhibit high levels of ubiquitination and that local signalling pathways trigger the ubiquitination and degradation of RhoA, a mediator of Sema3A-induced growth cone collapse. Inhibition of RhoA degradation is sufficient to remove the protein-synthesis requirement for Sema3A-induced growth cone collapse. In addition to RhoA, we find that locally translated proteins are the main targets of the ubiquitin-proteasome system in growth cones. Thus, local protein degradation is a major feature of growth cones and creates a requirement for local translation to replenish proteins needed to maintain growth cone responses. Local translation is a mechanism that leads to spatially and temporally restricted protein expression in specific subcellular sites, including dendrites, spines and developing axons. During development, neurons extend axons that contain ribosomes and translational machinery, as well as a subset of cellular mRNAs, many of which are selectively enriched in growth cones [1] . Specific mRNAs are locally translated in growth cones in response to various axonal guidance cues and neurotrophins [2] , [3] , leading to the rapid production of proteins that mediate the morphological responses to these signalling molecules. Distinct axonally localized transcripts have been linked to the action of both attractive and repulsive guidance cues. One of the first examples of local translation was shown in studies of Sema3A-induced growth cone collapse [4] . Sema3A induces the translation of axonally localized transcripts encoding RhoA, a small monomeric GTPase that induces depolymerization of F-actin [5] . Selective depletion of RhoA transcripts from axons markedly impairs Sema3A-induced growth cone collapse, linking local RhoA synthesis to the actions of Sema3A [6] . Similarly, other transcripts such as β-actin , cofilin and Par3 are locally translated in response to other guidance cues [7] , [8] , [9] , [10] . One puzzling aspect of local synthesis is why only a select subset of transcripts is translated in distal axons. Indeed, many signalling proteins are found in axons, but only a few of them are locally synthesized [3] , [11] . The remaining proteins are synthesized in the cell body and trafficked into axons. In the present study, we examine the basis for the requirement for local translation of RhoA in Sema3A-induced growth cone collapse. We find that growth cones are enriched in ubiquitination and proteasomal degradation, which is elicited by growth cone signalling pathways. In the case of NGF signalling, we show that the E3 ubiquitin ligase Smurf1 ubiquitinates and targets RhoA for local degradation. Preventing RhoA degradation blocks the requirement for local translation in Sema3A-induced growth cone collapse. In addition to RhoA, we find that locally translated proteins are frequently targeted by the ubiquitin-proteasome system (UPS) in growth cones. These findings demonstrate that local protein synthesis and degradation are highly coupled in growth cones, and reveal that local RhoA synthesis is required to replenish RhoA that is degraded as a result of growth cone signalling. Continuous need for local translation in Sema3A response To understand the basis for the selective synthesis of specific proteins in axons, we focused on Sema3A-induced growth cone collapse. This is one of the earliest and most widely used assays for the analysis of local translation [4] , [5] , [6] , [12] , [13] , [14] , [15] . Sema3A induces intra-axonal synthesis of RhoA, which is required to mediate morphological responses of growth cones to Sema3A [5] . As exposure to Sema3A induces RhoA synthesis, we wondered if the newly synthesized RhoA removes the requirement for further RhoA synthesis in subsequent exposures to Sema3A. To determine whether local protein synthesis is required in growth cones that have already been exposed to Sema3A, we first characterized the time course of Sema3A-induced growth cone collapse and recovery after removal of Sema3A. Embryonic day 14–15 (E14–15) rat dorsal root ganglion (DRG) neurons were cultured in compartmentalized microfluidic chambers [16] ( Supplementary Fig. 1a ). In these devices, axons grow through a 450-μm microgroove barrier and appear in the axonal compartment by 2 days in vitro (DIV2) [7] . The axonal and cell body compartments are fluidically isolated, which allows Sema3A to be applied selectively to axons without affecting cell bodies [7] , [16] . To monitor growth cone responses to Sema3A, individual growth cones were selected at the beginning of the experiment and monitored for the duration of the entire experiment ( Fig. 1a,b and Supplementary Fig. 1b ). Treatment of axons with Sema3A causes nearly maximal levels of growth cone collapse within 10 min of Sema3A application ( Fig. 1b ). As previously shown [4] , [5] , [12] , this collapse is protein synthesis dependent as it is blocked by application of the protein synthesis inhibitor anisomycin (40 μM; Supplementary Fig. 1c ). 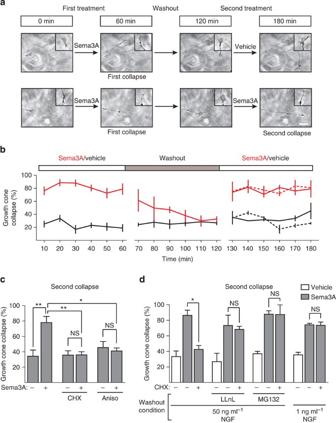Figure 1: The UPS and NGF maintain the local protein synthesis dependence of Sema3A-induced growth cone collapse. (a) Growth cones can undergo sequential rounds of Sema3A-induced growth cone collapse. Representative phase images of the same growth cones att=0 min (before any treatment),t=60 min (after 1 h of Sema3A or vehicle exposure),t=120 min (after washout) andt=180 min (after 1 h of the second Sema3A or vehicle treatment). Scale bar represents 5 μm. The insets show magnified images of the growth cones. (b) Quantification of results ina. The red line represents growth cones exposed to 450 ng ml−1Sema3A, whereas the black line represents vehicle-treated growth cones. In the last hour of the experiment (right side), the dashed red line indicates growth cones that were treated with vehicle in the first hour and Sema3A in the final hour, whereas the solid red line represents growth cones that had been exposed to Sema3A in the first hour and were again exposed to Sema3A in the final hour of the experiment. Growth cones treated with vehicle during the final hour are indicated with a black line (dashed for vehicle-treated during the first hour, solid for Sema3A-treated during the first hour).n≥15 growth cones per time point from at least three independent experiments. (c) The second Sema3A-induced growth cone collapse is dependent on local protein synthesis. Treatment of growth cones with the protein synthesis inhibitors cycloheximide (CHX, 10 μM) or anisomycin (Aniso, 40 μM) abolished the second Sema3A-induced growth cone collapse. **P<0.01, one-way analysis of variance (ANOVA) with Tukey’s multiple comparison test,n≥38 growth cones per condition from at least three independent experiments. (d) The requirement of local protein synthesis in Sema3A-induced growth cone collapse depends on UPS activity and NGF levels during washout. Addition of proteasome inhibitors (50 μM LLnL or 5 μM MG132) during the washout phase or washout in media containing minimal NGF concentrations (1 ng ml−1) rendered the second collapse protein synthesis independent. *P<0.05, one-way ANOVA with Tukey’s multiple comparison test,n≥34 growth cones per condition from at least three independent experiments. NS, not significant. Figure 1: The UPS and NGF maintain the local protein synthesis dependence of Sema3A-induced growth cone collapse. ( a ) Growth cones can undergo sequential rounds of Sema3A-induced growth cone collapse. Representative phase images of the same growth cones at t =0 min (before any treatment), t =60 min (after 1 h of Sema3A or vehicle exposure), t =120 min (after washout) and t =180 min (after 1 h of the second Sema3A or vehicle treatment). Scale bar represents 5 μm. The insets show magnified images of the growth cones. ( b ) Quantification of results in a . The red line represents growth cones exposed to 450 ng ml −1 Sema3A, whereas the black line represents vehicle-treated growth cones. In the last hour of the experiment (right side), the dashed red line indicates growth cones that were treated with vehicle in the first hour and Sema3A in the final hour, whereas the solid red line represents growth cones that had been exposed to Sema3A in the first hour and were again exposed to Sema3A in the final hour of the experiment. Growth cones treated with vehicle during the final hour are indicated with a black line (dashed for vehicle-treated during the first hour, solid for Sema3A-treated during the first hour). n ≥15 growth cones per time point from at least three independent experiments. ( c ) The second Sema3A-induced growth cone collapse is dependent on local protein synthesis. Treatment of growth cones with the protein synthesis inhibitors cycloheximide (CHX, 10 μM) or anisomycin (Aniso, 40 μM) abolished the second Sema3A-induced growth cone collapse. ** P <0.01, one-way analysis of variance (ANOVA) with Tukey’s multiple comparison test, n ≥38 growth cones per condition from at least three independent experiments. ( d ) The requirement of local protein synthesis in Sema3A-induced growth cone collapse depends on UPS activity and NGF levels during washout. Addition of proteasome inhibitors (50 μM LLnL or 5 μM MG132) during the washout phase or washout in media containing minimal NGF concentrations (1 ng ml −1 ) rendered the second collapse protein synthesis independent. * P <0.05, one-way ANOVA with Tukey’s multiple comparison test, n ≥34 growth cones per condition from at least three independent experiments. NS, not significant. Full size image We first asked whether growth cone collapse is reversible. After 1 h of Sema3A treatment, the axonal compartment was replaced with Sema3A-free media (‘washout’). Growth cone collapse returned to baseline levels within 1 h ( Fig. 1b ), indicating that growth cones exhibit morphologic recovery within 1 h of removing Sema3A. Next, we asked if growth cones that had been previously collapsed with Sema3A could respond to Sema3A again. After the 1-h recovery period, axons were again treated with Sema3A and the same growth cones were monitored for collapse. Growth cones that had previously collapsed upon first exposure to Sema3A underwent a second round of Sema3A-induced collapse that was similar in magnitude and kinetics to the collapse of growth cones naïve to Sema3A ( Fig. 1b ). As Sema3A induces local RhoA synthesis [5] , we wondered whether a subsequent treatment with Sema3A still requires local translation to induce growth cone collapse. To test this, we treated growth cones with Sema3A, allowed the collapsed growth cones to recover and then treated the growth cones with Sema3A for a second time. As with the first collapse, we found that protein synthesis inhibitors blocked the second collapse ( Fig. 1c and Supplementary Fig. 1d ). This indicates that the requirement for local translation persists even after proteins were synthesized by previous treatment of growth cones with Sema3A. NGF and the UPS confer protein synthesis dependence We next sought to understand the mechanism by which axons maintain the requirement for local protein synthesis in Sema3A-induced growth cone collapse. We speculated that the requirement for protein synthesis during the second round of collapse was due to the degradation of the protein that was locally synthesized during the first round of collapse. We therefore assayed the role of the UPS with proteasome inhibitors. Proteasome inhibitors stabilize proteins that are normally degraded via the UPS. They prevent ubiquitinated proteins from being degraded, thereby sequestering the ubiquitin monomers that would otherwise be released from protein-ubiquitin conjugates. As a result, proteins that would become ubiquitinated remain unmodified [17] . Thus, proteasome inhibition is a powerful approach to stabilize the levels of proteins that are normally targeted to the proteasome [18] . We tested whether the UPS was needed to maintain the local translation requirement for Sema3A-induced growth cone collapse. DIV3 DRG neurons were cultured in microfluidic chambers and Sema3A was applied to the axonal compartment. After the first round of collapse, axons were switched to Sema3A-free media, which contained either vehicle or proteasome inhibitors N-acetyl- L -leucyl-L-leucyl-L-norleucinal (LLnL; 50 μM) or MG132 (5 μM), and growth cones were allowed to recover for 1 h. The experimental treatments did not significantly affect morphological recovery of growth cones ( Supplementary Fig. 1e ). Growth cones that had recovered were subsequently analysed for protein synthesis dependence of growth cone collapse. For axons that were treated with vehicle during the recovery period, growth cone collapse remained protein synthesis dependent ( Fig. 1d ). However, in axons that were treated with proteasome inhibitors during the recovery period, growth cone collapse was no longer protein synthesis dependent ( Fig. 1d ). These experiments indicate that protein degradation is needed to maintain the protein synthesis dependence of Sema3A-induced growth cone collapse. To further understand the role of local degradation in mediating the requirement for local translation in axons, we tested whether pretreatment of axons with proteasomal inhibitors blocks the requirement for local translation in the initial exposure of axons to Sema3A. Indeed, treatment of DRG axons with MG132 (5 μM) for 1.5 h rendered Sema3A-induced growth cone collapse protein synthesis independent ( Supplementary Fig. 1f ). This effect was also seen in E17 rat hippocampal axons, suggesting that this mechanism is not limited to one neuronal cell type ( Supplementary Fig. 1g ). These data further support the idea that proteasomal degradation accounts for the requirement for local protein synthesis in Sema3A-induced growth cone collapse. The standard culture media for DRG neurons contain NGF, a trophic factor and one of the physiological guidance molecules for DRG neurons [19] , [20] . We wondered if NGF contributes to the protein synthesis dependence of Sema3A-induced growth cone collapse. As before, axons were treated with Sema3A for 1 h and then switched to Sema3A-free media to recover. The recovery media contained either minimal NGF (1 ng ml −1 ) or standard NGF (50 ng ml −1 ). After 1 h, growth cones exhibited similar morphological recovery, regardless of the recovery media ( Supplementary Fig. 1e ). In axons that recovered in standard culture media, Sema3A-induced growth cone collapse remained protein synthesis dependent. However, axons that recovered in media with minimal NGF exhibited collapse that was no longer protein synthesis dependent ( Fig. 1d ). Taken together, these data indicate that both proteasomal activity and NGF during the recovery phase lead to the dependence for local protein synthesis in Sema3A-induced growth cone collapse. NGF induces ubiquitination in growth cones Because both NGF signalling and the UPS establish the protein synthesis requirement for Sema3A-induced growth cone collapse, we wondered whether NGF mediates its effects, although the UPS. To test this possibility, we first asked if local NGF signalling involves the UPS by analysing NGF-induced axon outgrowth. In these experiments, dissociated DRG neurons were cultured in microfluidic chambers. After 3 DIV, the media in both the axonal and the cell body compartments were replaced with media containing a minimal concentration of NGF (1 ng ml −1 ) for 16 h to reduce axonal growth rates [7] . Axons were then incubated with either 0 or 50 ng ml −1 of NGF and the axon growth rate over 1 h was determined. Consistent with previous reports [7] , [21] , axonal application of NGF resulted in a twofold increase in the axonal growth rate relative to vehicle ( Fig. 2a–c ). Selective axonal application of two distinct proteasome inhibitors, lactacystin (10 μM) or LLnL (50 μM), markedly reduced NGF-stimulated axonal outgrowth without affecting basal axonal growth rates ( Fig. 2b,c ). These data indicate that NGF-stimulated outgrowth utilizes intra-axonal UPS activity. 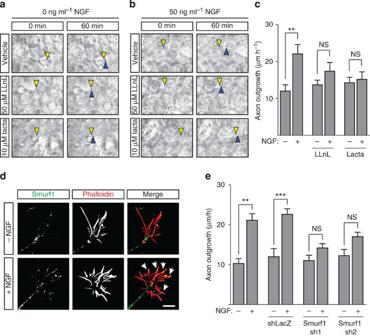Figure 2: NGF signalling induces local recruitment of the UPS via Smurf1. (a,b) NGF-dependent axon outgrowth requires the UPS. Axonal application of NGF leads to a significant increase in the rate of axon outgrowth that is abolished by treatment of axons with the proteasome inhibitors LLnL (50 μM) or lactacystin (10 μM). Phase images show representative axons att=0 andt=60 min after exposure to no NGF (a) or 50 ng ml−1NGF (b). The yellow triangles indicate the position of the growth cone at the beginning of the experiment (t=0 min), whereas the blue triangles indicate the position of the growth cone at the end of the experiment (t=60 min). Scale bar represents 10 μm. (c) Quantification of results ina,b. Axon growth was calculated by measuring the distance travelled by the growth cone betweent=0 andt=60 min. **P<0.01, one-way analysis of variance (ANOVA) with Tukey’s multiple comparison test,n≥71 axons per condition from at least three independent experiments. (d) Smurf1 levels and localization within growth cones change upon NGF treatment. DIV3–4 rat DRG neurons were exposed to 0 or 50 ng ml−1of NGF for 10 min, followed by fixation and staining. Immunofluorescence images of endogenous Smurf1 (green) and Alexa-568-phalloidin (red) show that exposure to NGF increases the amount of Smurf1 in growth cones, with more Smurf1 localizing to filopodia (white arrows). (e) Smurf1 is required for NGF-induced axon outgrowth. NGF-induced axon outgrowth is abolished in Smurf1 knockdown cells compared with wild-type or shLacZ controls. The basal growth rate is not affected by Smurf1 knockdown. **P<0.01, ***P<0.001, one-way ANOVA with Tukey’s multiple comparison tests,n≥87 axons per condition from at least three independent experiments. NS, not significant. Figure 2: NGF signalling induces local recruitment of the UPS via Smurf1. ( a , b ) NGF-dependent axon outgrowth requires the UPS. Axonal application of NGF leads to a significant increase in the rate of axon outgrowth that is abolished by treatment of axons with the proteasome inhibitors LLnL (50 μM) or lactacystin (10 μM). Phase images show representative axons at t =0 and t =60 min after exposure to no NGF ( a ) or 50 ng ml −1 NGF ( b ). The yellow triangles indicate the position of the growth cone at the beginning of the experiment ( t =0 min), whereas the blue triangles indicate the position of the growth cone at the end of the experiment ( t =60 min). Scale bar represents 10 μm. ( c ) Quantification of results in a , b . Axon growth was calculated by measuring the distance travelled by the growth cone between t =0 and t =60 min. ** P <0.01, one-way analysis of variance (ANOVA) with Tukey’s multiple comparison test, n ≥71 axons per condition from at least three independent experiments. ( d ) Smurf1 levels and localization within growth cones change upon NGF treatment. DIV3–4 rat DRG neurons were exposed to 0 or 50 ng ml −1 of NGF for 10 min, followed by fixation and staining. Immunofluorescence images of endogenous Smurf1 (green) and Alexa-568-phalloidin (red) show that exposure to NGF increases the amount of Smurf1 in growth cones, with more Smurf1 localizing to filopodia (white arrows). ( e ) Smurf1 is required for NGF-induced axon outgrowth. NGF-induced axon outgrowth is abolished in Smurf1 knockdown cells compared with wild-type or shLacZ controls. The basal growth rate is not affected by Smurf1 knockdown. ** P <0.01, *** P <0.001, one-way ANOVA with Tukey’s multiple comparison tests, n ≥87 axons per condition from at least three independent experiments. NS, not significant. Full size image We then tested if NGF induces ubiquitination in growth cones by monitoring the appearance of ubiquitin conjugates in growth cones. DIV3 DRG explants were cultured in media containing 1 ng ml −1 of NGF for 16 h to reduce baseline NGF signalling. Cultures were then treated with either 0 or 50 ng ml −1 NGF for 10 min and immunostained using linkage-specific polyubiquitin antibodies [22] . In these experiments, MG132 (5 μM) was included to prevent turnover of newly ubiquitinated proteins. Immunostaining with antibodies specific for lysine 48 (K48)-linked polyubiquitin chains, which is found on proteins that are targeted for proteasomal degradation [23] , revealed a significant increase of K48-linked ubiquitin conjugates in growth cones after 10 min of NGF treatment ( Supplementary Fig. 2a,b ). In contrast, NGF exposure did not increase K63-linked ubiquitin chains ( Supplementary Fig. 2b ), which are thought to be a marker for ubiquitin-dependent non-degradation pathways [23] . Together, these data suggest that NGF signalling recruits the UPS and induces K48-linked polyubiquitination in growth cones. Smurf1 mediates NGF signalling in growth cones To determine how NGF signalling influences the requirement for local protein synthesis in axons, we sought to identify the E3 ubiquitin ligase that mediates the effects of NGF. We considered the possibility that NGF induces ubiquitination through Smurf1, a HECT E3 ubiquitin ligase. In epithelial cells, recruitment of Smurf1 induces actin polymerization and cellular protrusions [24] , [25] , which are reminiscent of NGF-induced actin-rich filipodia [26] . Smurf1 is also expressed in neurons and has been shown to contribute to axon specification from immature neurites [27] . We therefore tested whether NGF signalling in axons utilizes Smurf1. To address this, we first examined Smurf1 localization in growth cones. DIV3 DRG neurons were cultured in minimal NGF (1 ng ml −1 ) for 16 h and then treated with 50 ng ml −1 of NGF for 10 min. Smurf1 localization was determined by immunofluorescence. NGF treatment led to an increase in the level of Smurf1, which was detected within growth cones and along filopodia ( Fig. 2d and Supplementary Fig. 2c–e ). Similarly, NGF treatment led to a subtle relocalization of a Cherry-Smurf1 reporter expressed in dissociated E14 DRG neurons, with occasional Smurf1 fluorescent puncta observed trafficking to the base of emerging or elongating filopodia ( Supplementary Movie 1 and Supplementary Fig. 2f ). Although alteration of Smurf1 localization does not definitively link Smurf1 to NGF signalling, it suggests a potential role for Smurf1 at sites of NGF-induced actin remodelling. Taken together, these data reveal Smurf1 localization in filopodia and raise the possibility that NGF treatment may affect Smurf1 localization to influence growth cone morphology. We next asked whether Smurf1 mediates NGF signalling by monitoring the effect of Smurf1 knockdown on NGF-induced outgrowth. In these experiments, we used a microfluidic chamber with longer microgrooves (1,500 μm). This was necessary because the neurons needed to be cultured for 5 days for knockdown to occur ( Supplementary Fig. 3a ), and at this time point, the axons are too long for the standard microfluidic chamber. DRG neurons were transduced upon plating with lentiviral constructs expressing either of two Smurf1-specific small hairpin RNA (shRNAs; Supplementary Fig. 3b,c ). Axons reached the distal compartment by DIV4–5, at which point NGF-induced outgrowth was monitored. Wild-type neurons and neurons infected with control LacZ-specific shRNA (shLacZ) exhibited a twofold increase in axonal growth upon application of NGF to the distal compartment. However, this increase was abolished in neurons expressing Smurf1-specific shRNAs ( Fig. 2e ). These data suggest that Smurf1 mediates the local effects of NGF on axonal growth. We next wanted to determine whether Smurf1 has a more general role in regulating axonal growth. Another system used to monitor axon growth involves the growth of dorsal spinal commissural axons towards the spinal midline, which is regulated, in part, by netrin-1 (ref. 28 ). E10.5 mouse spinal cord explants were electroporated with a plasmid expressing a dominant-negative Smurf1 construct (Smurf1 C699A) [29] . After 48 h, dorsal commissural neurons expressing Smurf1 C699A exhibited impaired axonal outgrowth towards the spinal midline ( Supplementary Fig. 3d–f ). Taken together, these data support the idea that Smurf1 contributes to pathways that promote axonal growth. Smurf1 confers the requirement for protein synthesis Our data linking the E3 ubiquitin ligase Smurf1 to NGF signalling prompted us to ask if Smurf1 mediates the proteasome-dependent protein degradation that leads to the requirement for protein synthesis in Sema3A-induced growth cone collapse. To test this, E15 DRG neurons were cultured in microfluidic chambers and infected with lentiviral constructs expressing either Smurf1-specific shRNAs or the control shLacZ. In neurons expressing shLacZ, Sema3A-induced growth cone collapse was protein synthesis dependent ( Fig. 3a and Supplementary Fig. 4a ). However, in neurons lacking Smurf1, Sema3A-induced growth cone collapse was no longer protein synthesis dependent ( Fig. 3a and Supplementary Fig. 4a ). Similarly, Sema3A-induced growth cone collapse was no longer protein synthesis dependent in neurons expressing the dominant negative Smurf1 C699A [29] ( Fig. 3b and Supplementary Fig. 4b ). These data indicate that Smurf1 confers the local translation requirement for Sema3A-induced collapse in sensory axons. 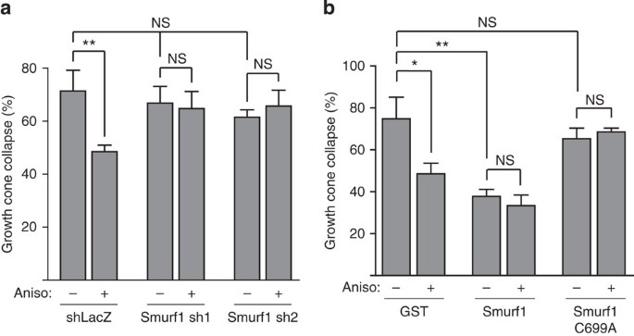Figure 3: Smurf1 maintains the protein synthesis requirement in Sema3A-induced growth cone collapse. (a) Smurf1 accounts for the protein synthesis dependence of Sema3A-induced growth cone collapse. Rat DRG neurons were transduced upon plating with lentiviral constructs expressing two distinct Smurf1 shRNAs or a control non-targeting shRNA (shLacZ) and grown for 5 DIV. Application of anisomycin (Aniso, 40 μM) reduced Sema3A-induced growth cone collapse in neurons expressing shLacZ but not in Smurf1 knockdown neurons. **P<0.01, one-way analysis of variance (ANOVA) with Tukey’s multiple comparison test,n≥58 growth cones per condition from at least three independent experiments. (b) Overexpression of a catalytically inactive mutant form of Smurf1 (Smurf1 C699A) leads to a Sema3A-induced growth cone collapse that is protein synthesis independent. GST, Glutathione S-Transferase. *P<0.05, **P<0.01, one-way ANOVA with Tukey’s multiple comparison test,n≥53 growth cones per condition from at least three independent experiments. NS, not significant. Figure 3: Smurf1 maintains the protein synthesis requirement in Sema3A-induced growth cone collapse. ( a ) Smurf1 accounts for the protein synthesis dependence of Sema3A-induced growth cone collapse. Rat DRG neurons were transduced upon plating with lentiviral constructs expressing two distinct Smurf1 shRNAs or a control non-targeting shRNA (shLacZ) and grown for 5 DIV. Application of anisomycin (Aniso, 40 μM) reduced Sema3A-induced growth cone collapse in neurons expressing shLacZ but not in Smurf1 knockdown neurons. ** P <0.01, one-way analysis of variance (ANOVA) with Tukey’s multiple comparison test, n ≥58 growth cones per condition from at least three independent experiments. ( b ) Overexpression of a catalytically inactive mutant form of Smurf1 (Smurf1 C699A) leads to a Sema3A-induced growth cone collapse that is protein synthesis independent. GST, Glutathione S-Transferase. * P <0.05, ** P <0.01, one-way ANOVA with Tukey’s multiple comparison test, n ≥53 growth cones per condition from at least three independent experiments. NS, not significant. Full size image NGF induces RhoA ubiquitination via Smurf1 We next sought to determine the targets downstream of NGF-dependent Smurf1 signalling that confer the protein synthesis requirement to Sema3A-induced growth cone collapse. Smurf1 has been shown to directly ubiquitinate and trigger the degradation of RhoA in diverse cell types [24] , [25] , [27] , [29] . We therefore first addressed whether NGF can induce RhoA ubiquitination. Treatment of undifferentiated PC12 cells with NGF resulted in the rapid appearance of ubiquitinated RhoA within 10 min ( Fig. 4a ). We next asked if NGF induces RhoA degradation in growth cones of DRG neurons. To test this, we incubated DIV3 rat E14 DRG neurons in media containing minimal NGF (1 ng ml −1 ) for 18 h to reduce NGF signalling. Neurons were then treated with 50 ng ml −1 NGF or NGF plus MG132 (5 μM) for 20 or 60 min and RhoA levels in growth cones were quantified by immunofluorescence. NGF treatment led to a significant decrease in RhoA levels in growth cones in 60 min, which was prevented by co-application of the proteasome inhibitor MG132 ( Fig. 4b,c and Supplementary Fig. 5a ). These data indicate that NGF signalling leads to RhoA degradation via the UPS. 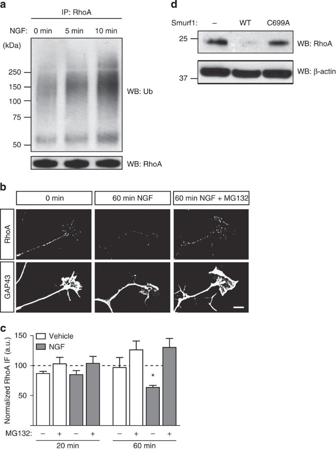Figure 4: Smurf1 degradation of RhoA leads to the protein synthesis requirement in Sema3A-induced growth cone collapse. (a) NGF induces rapid ubiquitination of endogenous RhoA in PC12 cells. PC12 cells were exposed to NGF (100 ng ml−1) for the indicated times. Endogenous RhoA was immunoprecipitated (IP) with an anti-RhoA antibody and the degree of ubiquitination was evaluated by western blot (WB) analysis with an anti-ubiquitin antibody. (b) NGF induces proteasomal-mediated degradation of endogenous RhoA in growth cones of DRG neurons. Neurons were incubated in minimal NGF (1 ng ml−1) for 18 h to decrease NGF signalling. DRG neurons were then exposed to either 0 or 50 ng ml−1of NGF either in the presence (NGF+MG132) or absence of MG132 (5 μM) for the indicated times, and fixed and stained to quantify the levels of endogenous RhoA within growth cones. Scale bar represents 10 μm. (c) Quantification of results inb. RhoA levels were normalized to the levels at 0 min (dotted line). For quantification purposes, the RhoA immunofluorescence signal was normalized to that of GAP43. *P<0.05, one-way analysis of variance,n≥35 per condition from at least three independent experiments. (d) Smurf1 induces degradation of endogenous RhoA. RhoA levels were determined in untransfected cells (−) and in cells expressing wild-type Smurf1 (WT) or a catalytically inactive mutant form of Smurf1 (Smurf1 C699A). Figure 4: Smurf1 degradation of RhoA leads to the protein synthesis requirement in Sema3A-induced growth cone collapse. ( a ) NGF induces rapid ubiquitination of endogenous RhoA in PC12 cells. PC12 cells were exposed to NGF (100 ng ml −1 ) for the indicated times. Endogenous RhoA was immunoprecipitated (IP) with an anti-RhoA antibody and the degree of ubiquitination was evaluated by western blot (WB) analysis with an anti-ubiquitin antibody. ( b ) NGF induces proteasomal-mediated degradation of endogenous RhoA in growth cones of DRG neurons. Neurons were incubated in minimal NGF (1 ng ml −1 ) for 18 h to decrease NGF signalling. DRG neurons were then exposed to either 0 or 50 ng ml −1 of NGF either in the presence (NGF+MG132) or absence of MG132 (5 μM) for the indicated times, and fixed and stained to quantify the levels of endogenous RhoA within growth cones. Scale bar represents 10 μm. ( c ) Quantification of results in b . RhoA levels were normalized to the levels at 0 min (dotted line). For quantification purposes, the RhoA immunofluorescence signal was normalized to that of GAP43. * P <0.05, one-way analysis of variance, n ≥35 per condition from at least three independent experiments. ( d ) Smurf1 induces degradation of endogenous RhoA. RhoA levels were determined in untransfected cells (−) and in cells expressing wild-type Smurf1 (WT) or a catalytically inactive mutant form of Smurf1 (Smurf1 C699A). Full size image We then asked if Smurf1 mediates the ubiquitination of RhoA. Expression of Smurf1 in HEK293 cells led to accumulation of polyubiquitinated forms of RhoA ( Supplementary Fig. 5b ). Smurf1 expression resulted in a marked reduction in RhoA levels, whereas RhoA levels were unaffected following expression of the catalytically inactive C699A Smurf1 mutant ( Fig. 4d and Supplementary Fig. 5c ). Moreover, Smurf1 knockdown prevented NGF-induced RhoA ubiquitination ( Supplementary Fig. 5d ). To determine whether Smurf1 regulates RhoA levels in axons, we quantified RhoA levels in DRG growth cones following lentiviral expression of a Smurf1-specific shRNA. We found that Smurf1 knockdown increased growth cone levels of RhoA compared with control ( Supplementary Fig. 5e ). Together, these results suggest that Smurf1 catalyses the degradation of RhoA. Smurf1 ubiquitinates RhoA at Lys 6, 7 and 51 We sought to generate a ubiquitination-resistant form of RhoA. Previously, RhoA lysine 6 and lysine 7 were shown to be ubiquitinated by Smurf1 (ref. 25 ). However, mutation of these two lysines (K6/7R) did not substantially prevent Smurf1-induced RhoA degradation ( Fig. 5a and Supplementary Fig. 6a ). We therefore wondered if ubiquitination of additional lysines may contribute to Smurf1-mediated RhoA degradation. Examination of the crystal structure of RhoA (PDB: 2A3B) indicates that an additional lysine residue, K51, is in close proximity to K6 and K7 ( Fig. 5b ), and therefore may also be targeted by the E3 ubiquitin ligase that transfers ubiquitin to the surface of RhoA when lysines 6 and 7 are mutated to arginine. Indeed, the triple mutant of RhoA, K6/7/51R, displays reduced ubiquitination levels compared with RhoA or RhoA K6/7R ( Supplementary Fig. 6b ). We thus tested the susceptibility of RhoA K6/7/51R to Smurf1-mediated degradation. We found that this mutant was no longer susceptible to degradation when co-expressed with Smurf1 ( Fig. 5a ), indicating that Smurf1 mediates degradation of RhoA mainly through these residues. 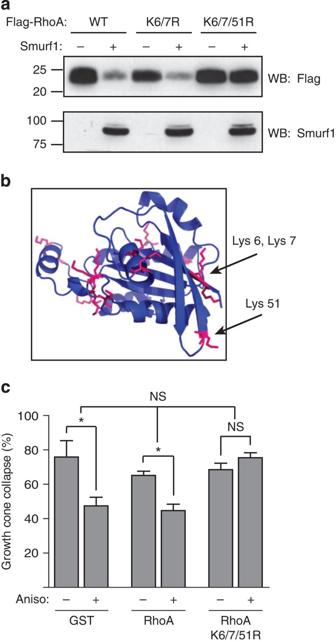Figure 5: Smurf1 ubiquitinates RhoA at Lys 6, 7 and 51. (a) RhoA is degraded by Smurf1 through ubiquitination of Lys 6, 7 and 51. Flag-tagged wild-type or mutant RhoA-expressing plasmids were co-transfected with GFP- or Smurf1-expressing plasmids in HEK293T cells using calcium phosphate transfection. (b) RhoA Lys 6, 7 and 51 are in close proximity in the crystal structure. The three-dimensional structure of RhoA (PDB: 2A3B) showed that Lys 51 is positioned near Lys 6 and 7 (black arrows) on the same surface. Lysines are indicated in magenta while the rest of the protein is in blue. (c) RhoA degradation is required to maintain the protein synthesis dependence of Sema3A-induced growth cone collapse. Sema3A-induced growth cone collapse was evaluated in neurons expressing GST (GST), wild-type (WT) RhoA (RhoA) or the K6/7/51R mutant form of RhoA (K6/7/51R). The samples were treated with Sema3A (450 ng ml−1) and with DMSO or anisomycin (40 μM). *P<0.05, one-way analysis of variance with Tukey’s multiple comparison test,n≥51 growth cones per condition from at least three independent experiments. WB, western blot. Figure 5: Smurf1 ubiquitinates RhoA at Lys 6, 7 and 51. ( a ) RhoA is degraded by Smurf1 through ubiquitination of Lys 6, 7 and 51. Flag-tagged wild-type or mutant RhoA-expressing plasmids were co-transfected with GFP- or Smurf1-expressing plasmids in HEK293T cells using calcium phosphate transfection. ( b ) RhoA Lys 6, 7 and 51 are in close proximity in the crystal structure. The three-dimensional structure of RhoA (PDB: 2A3B) showed that Lys 51 is positioned near Lys 6 and 7 (black arrows) on the same surface. Lysines are indicated in magenta while the rest of the protein is in blue. ( c ) RhoA degradation is required to maintain the protein synthesis dependence of Sema3A-induced growth cone collapse. Sema3A-induced growth cone collapse was evaluated in neurons expressing GST (GST), wild-type (WT) RhoA (RhoA) or the K6/7/51R mutant form of RhoA (K6/7/51R). The samples were treated with Sema3A (450 ng ml −1 ) and with DMSO or anisomycin (40 μM). * P <0.05, one-way analysis of variance with Tukey’s multiple comparison test, n ≥51 growth cones per condition from at least three independent experiments. WB, western blot. Full size image RhoA degradation maintains the need for protein synthesis We next asked if Smurf1-mediated degradation of RhoA accounts for the local synthesis requirement of growth cone collapse. To test this, we monitored Sema3A-induced growth cone collapse in neurons expressing the ubiquitination-resistant RhoA mutant (K6/7/51R). This RhoA mutant is still enzymatically active as assessed by its ability to induce stress fibre formation in fibroblasts [30] ( Supplementary Fig. 6c,d ). E15 DRG neurons were transduced with lentiviral constructs expressing GFP-GST, GFP-RhoA or GFP-RhoA K6/7/51R and tested for protein synthesis-dependent growth cone collapse in media containing 50 ng ml −1 NGF. In GFP-GST- or GFP-RhoA-expressing sensory neurons, Sema3A-induced growth cone collapse was protein synthesis dependent ( Fig. 5c ). However, in neurons expressing RhoA K6/7/51R Sema3A-induced growth cone collapse was no longer protein synthesis dependent ( Fig. 5c and Supplementary Fig. 6e ). These data suggest that Smurf1-mediated degradation of RhoA maintains the requirement for local translation in Sema3A-induced growth cone collapse. High levels of UPS components in growth cones The finding that RhoA is locally degraded made us wonder if local degradation is a general mechanism used by growth cones. To test this idea, we immunostained low-density DIV4 DRG cultures with the K48-Ub-specific antibody. In these experiments, we used neurons grown under normal culturing conditions, rather than NGF-deprived neurons, as in Supplementary Fig. 2a , and did not include MG132. We found that growth cones contained high levels of K48-Ub conjugates ( Fig. 6a and Supplementary Fig. 7a ). Within growth cones, immunostaining frequently showed a polarized distribution, with maximal signals within filopodia ( Fig. 6a , inset). 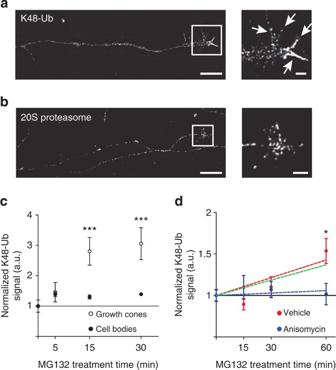Figure 6: Growth cones exhibit a high degree of ubiquitination and protein turnover. (a) Growth cones display high levels of ubiquitination. DRG neurons cultured in standard growth conditions were immunostained with K48-linkage-specific polyubiquitin antibody (K48-Ub). The white arrows in the inset indicate the filopodia. Scale bar represents 10 μm, inset scale bar represents 2 μm. (b) Growth cones are enriched in 20S proteasomal subunits, which primarily localize to the palm region of growth cones. DRG neurons were immunostained with an antibody recognizing the 20S proteasome. Scale bar represents 10 μm, inset scale bar represents 2 μm. (c) Growth cone proteins are rapidly ubiquitinated. DRG neurons were treated with MG132 (5 μM) for the times indicated and stained for K48-Ub. The signal was normalized for volume by tau-1 staining and measured in growth cones (open circles) and cell bodies (closed circles). ***P<0.001, Student’st-test,n≥27 growth cones and cell bodies per condition per time point from at least three independent experiments. (d) Locally synthesized proteins are the primary target of ubiquitination in growth cones. DIV5 DRG axons were treated for the indicated times with MG132 and stained for K48-Ub. The immunofluorescence signal in growth cones was normalized to the average signal for vehicle-treated controls. Red and blue circles indicate treated with vehicle or anisomycin (40 μM), respectively. The ubiquitination of the locally translated pool of proteins (green line) can be extrapolated by subtracting the ubiquitination rate of the cell body-derived pool (blue line, linear regression) from the total axonal protein pool (red line, linear regression). The locally synthesized protein pool accounts for the majority of the ubiquitination seen in axonal growth cones. *P<0.05, Student’st-test,n≥26 growth cones per condition from at least three independent experiments. Figure 6: Growth cones exhibit a high degree of ubiquitination and protein turnover. ( a ) Growth cones display high levels of ubiquitination. DRG neurons cultured in standard growth conditions were immunostained with K48-linkage-specific polyubiquitin antibody (K48-Ub). The white arrows in the inset indicate the filopodia. Scale bar represents 10 μm, inset scale bar represents 2 μm. ( b ) Growth cones are enriched in 20S proteasomal subunits, which primarily localize to the palm region of growth cones. DRG neurons were immunostained with an antibody recognizing the 20S proteasome. Scale bar represents 10 μm, inset scale bar represents 2 μm. ( c ) Growth cone proteins are rapidly ubiquitinated. DRG neurons were treated with MG132 (5 μM) for the times indicated and stained for K48-Ub. The signal was normalized for volume by tau-1 staining and measured in growth cones (open circles) and cell bodies (closed circles). *** P <0.001, Student’s t -test, n ≥27 growth cones and cell bodies per condition per time point from at least three independent experiments. ( d ) Locally synthesized proteins are the primary target of ubiquitination in growth cones. DIV5 DRG axons were treated for the indicated times with MG132 and stained for K48-Ub. The immunofluorescence signal in growth cones was normalized to the average signal for vehicle-treated controls. Red and blue circles indicate treated with vehicle or anisomycin (40 μM), respectively. The ubiquitination of the locally translated pool of proteins (green line) can be extrapolated by subtracting the ubiquitination rate of the cell body-derived pool (blue line, linear regression) from the total axonal protein pool (red line, linear regression). The locally synthesized protein pool accounts for the majority of the ubiquitination seen in axonal growth cones. * P <0.05, Student’s t -test, n ≥26 growth cones per condition from at least three independent experiments. Full size image To further assess the importance of the axonal UPS, we stained axons using an antibody for the 20S subunit of the proteasome. 20S was located throughout axons with the most prominent localization in the central region of growth cones ( Fig. 6b and Supplementary Fig. 7b ). The robust localization of K48-linked ubiquitin conjugates and 20S in growth cones suggests that the growth cone is a neuronal compartment that has a higher degree of proteasome-dependent protein turnover than the soma. To understand the significance of protein turnover in the growth cone, we asked how the rate of ubiquitination in growth cones compares to that in cell bodies. We treated DIV3 DRG neurons in culture with the proteasome inhibitor MG132 (5 μM) for different times, and measured accumulation of ubiquitin conjugates. Compared with cell bodies, K48-linked ubiquitin conjugates appeared at a markedly higher rate in growth cones ( Fig. 6c ). These data suggest that the growth cone has a higher rate of protein ubiquitination than other parts of the neuron. Differential stability of locally synthesized proteins Our findings suggest that growth cones exhibit a high degree of UPS-dependent protein turnover. In the case of RhoA, degradation is linked to NGF signalling, and is replenished for Sema3A signalling by local translation. However, it is not clear if other locally synthesized proteins are also subjected to local degradation in axons. Therefore, we asked if locally synthesized proteins are preferentially targeted for degradation compared with growth cone proteins that are transported from the cell body. To test this idea, we sought to determine the ubiquitination rate of locally synthesized proteins and cell body-derived proteins. To preferentially monitor the ubiquitination of cell body-derived proteins, we cultured DRG neurons in microfluidic chambers for 5 DIV and treated axons with anisomycin, which is expected to reduce the levels of locally synthesized proteins. As a control, we confirmed that this treatment does not affect the capacity for ubiquitination or proteasomal degradation in growth cones ( Supplementary Fig. 7c ). We then applied MG132 to axons to monitor the rate of ubiquitination of the remaining cell body-derived proteins. Immunofluorescence staining using antibodies that detect K48-linked ubiquitin conjugates revealed minimal accumulation of ubiquitinated proteins over 60 min ( Fig. 6d ). However, in axons that were not treated with anisomycin, and which therefore contained both locally synthesized and cell body-derived proteins, K48-linked ubiquitin conjugates markedly increased over the 60-min time course ( Fig. 6d ). We next extrapolated the rate of ubiquitination of locally synthesized proteins by subtracting the rate of ubiquitination in anisomycin-treated axons, which contain cell body-derived proteins, from that of vehicle-treated axons, which contain both locally synthesized and cell body-derived proteins ( Fig. 6d ). This analysis revealed that the rate of ubiquitination of locally synthesized proteins was substantially higher than that of cell body-derived proteins. These data suggest that locally synthesized proteins are preferentially targeted for local ubiquitination, whereas cell body-derived proteins are more stable and not major targets of the UPS in growth cones. Together, our data support a model in which the primary targets of the UPS in the growth cone are proteins that are being locally synthesized ( Supplementary Fig. 7d ). Local translation is required for the actions of diverse classes of axon guidance cues [31] . However, only a small subset of the axonal proteome is locally translated, and the basis for this selectivity is poorly understood. To shed light on this selectivity, we explored Sema3A-dependent synthesis of RhoA, which promotes growth cone collapse [5] . We find that RhoA levels in growth cones are regulated by both local translation and local degradation. We show that RhoA is unstable in axons due to NGF signalling, which promotes Smurf1-dependent proteasomal degradation of RhoA. However, because RhoA is needed for Sema3A-induced growth cone collapse, a source of RhoA is needed in order to reconstitute Sema3A signalling. Indeed, we show that blocking RhoA degradation removes the classical requirement for local protein synthesis in Sema3A-induced growth cone collapse. Thus, Sema3A likely has two independent functions in axon: first, it induces local translation of RhoA; and second, it activates growth cone-localized RhoA to promote growth cone collapse. Taken together, these findings suggest that local translation of RhoA is utilized as a mechanism to replenish RhoA that is locally degraded by the UPS. Our data indicate that growth cones exhibit high levels of ubiquitination and proteasomal degradation. Although ubiquitin-mediated protein degradation was initially thought to mediate the degradation of aged proteins, it is now recognized that the UPS is used by diverse signalling pathways, and typically involves highly selective protein degradation [32] . Notably, we observed a high degree of protein turnover in growth cones. However, when proteins are degraded during growth cone signalling, the proteins will need to be replenished. In the case of RhoA, local synthesis enables sufficient amounts of protein required for Sema3A signalling. The finding that the same proteins that are targeted by the UPS are also capable of being locally translated supports the idea that local translation and local degradation are highly coupled processes in growth cones. To our knowledge, this is the first time that the UPS and local translation have been linked to locally regulate the levels of proteins synthesized in distal axons. Another way to view our data is that the function of local degradation may be to terminate signalling pathways enabled by locally translated proteins. Because local translation may be important to transiently alter growth cone properties, mechanisms likely exist to end these pathways. Local degradation of locally translated proteins could thereby restore growth cones to a basal state. Coupled local translation and degradation may therefore also function to terminate local translation pathways. In addition to Smurf1, which degrades RhoA, other growth cone-localized E3 ligases may also target proteins that are locally synthesized. Indeed, neurites contain the E3 ligase Siah1 (ref. 33 ), which ubiquitinates and degrades Par3 (ref. 34 ). Par3 is locally synthesized in axons in response to NGF and netrin-1 treatment [7] . In addition, other E3 ubiquitin ligases have been found in growth cones of developing neurons, including RNF6 and Nedd4 (refs 35 , 36 ). Nedd4 has been linked to neurotrophin-dependent cell survival through its differential regulation of the neurotrophin receptors [37] . Transcripts encoding several protein targets of these E3 ligases, such as Notch and PTEN, have been identified in axonal libraries [1] , [38] , further supporting the idea that diverse locally translated proteins may be coupled to local degradation pathways. At present, only a few E3 ligases have been definitively localized to growth cones. This study uncovers a novel role for E3 ubiquitin ligases in developing axons, and points to the importance of identifying other E3 ubiquitin ligases that are localized to growth cones in order to understand the biological significance of local degradation and translation events. Although we find that local proteasomal degradation of RhoA leads to the local synthesis requirement for RhoA, other removal pathways may also lead to a requirement for local translation. Retrograde trafficking has been shown to deplete several proteins from axons, including importins, CREB and SMAD1/5/8 (refs 39 , 40 , 41 , 42 ). In the case of β-actin, N-terminal processing alters its polymerization properties [43] , [44] , which may necessitate continuous β-actin synthesis to obtain unmodified protein. Thus, local translation may be coupled to additional removal pathways besides proteasomal degradation. Our study identifies Smurf1 as an E3 ligase that promotes the protein-synthesis dependence of Sema3A-induced growth cone collapse. Smurf1 has been previously shown to regulate protrusion formation in epithelial cells [24] , [25] and has been implicated in axon specification from undifferentiated neurites in early stages of neuronal development [27] . We find that Smurf1 remains in axons after specification and has roles in mediating responses to guidance cues. Smurf1 is localized to growth cones, including filopodia and filopodial tips. The localization of Smurf1 may enable local RhoA degradation, which would lead to increased actin polymerization needed for filopodia formation at these sites. Thus, Smurf1 may influence actin-dependent processes in the growth cone, including axon outgrowth and growth cone collapse [45] , [46] . Our finding that Smurf1 activity reduces growth cone collapse and enhances axon outgrowth reflects the common role for actin dynamics in these processes [45] , [46] . Restoring RhoA levels would be critical for limiting axon outgrowth induced by Smurf1 activity. Although Smurf1 is highly expressed in neurons, the related E3 ubiquitin ligase Smurf2 can also degrade RhoA [47] , [48] . Smurf1 and Smurf2 appear to have redundant functions, as Smurf1 and Smurf2 null mice each exhibit minor phenotypes, whereas Smurf1 / Smurf2 double knockout mice display severe embryonic defects and lethality between E10.5 and E12.5 (ref. 49 ). Smurf2 as well as other pathways may therefore also contribute to RhoA regulation in growth cones. Although our studies relied on the widely used growth cone collapse assay, this assay likely has relevance to turning responses seen in response to repulsive guidance cues in vivo . Axonal turning responses may reflect collapse of the portion of the growth cone on the side of the axon closer to the source of the repulsive guidance cue. Indeed, turning responses of axons have been linked to asymmetric local protein synthesis across the growth cone [9] , [10] . The reciprocal regulation of axonal proteins by local synthesis and local degradation suggests an additional mechanism to achieve asymmetry through differential proteasomal degradation across the growth cone. Gradations in local synthesis as well as local degradation may thus allow growth cones to finely tune their response to guidance cue gradients. Microfluidic chamber assays To selectively apply treatments to distal axons and growth cones without affecting cell bodies, neurons were grown in microfluidic chambers (Xona Microfluidics) [7] . Chambers were assembled on glass coverslides or plastic dishes coated with 1 mg ml −1 poly-Lysine (Trevigen) and 3.33 μg ml −1 laminin (Cultrex, Trevigen). About 20,000 dissociated DRG neurons were plated per chamber. Axons typically start crossing to the other side on DIV2–3 in two-compartment chambers and by DIV4–5 in three-compartment chambers, and experiments were performed when at least 30% of the axonal compartment was populated by axons. Neuronal and PC12 cell cultures All reagents were purchased from Invitrogen unless otherwise specified. DRG neurons harvested from E14–15 Sprague–Dawley rat embryos [5] , [7] . All animal work was conducted according to the relevant national and international guidelines approved by the Institutional Animal Care and Use Committee. DRG neurons were dissected in L-15 and dissociated in TrypLE for 15 min before plating. Cells were grown in Neurobasal medium supplemented with B-27, glutamine (2 mM), 5-fluoro-2′-deoxyuridine (10 μM, Sigma), penicillin (100 IU), streptomycin (100 μg ml −1 ) and NGF (2.5S, 50 ng ml −1 ). For cells cultured in microfluidic chambers, the culturing medium was exchanged every 2 days or when required by the experiment (see below). Hippocampal neurons were harvested from E18 rat embryos as previously described [16] . Cells were plated in microfluidic devices at a concentration of ∼ 7 × 10 4 cells in 10 μl and grown for 5 DIV to allow axons to cross to the other side of the chamber in Neurobasal medium supplemented with B-27, glutamine, 5-fluoro-2′-deoxyuridine (10 μM, Sigma), Glutamax (2 mM), penicillin (100 IU ml −1 ) and streptomycin (100 μg ml −1 ). The medium was exchanged 24 h before the experiment with pre-equilibrated culture medium containing 25 μM brain-derived neurotrophic factor (BDNF). PC12 cells were cultured in DMEM containing 10% fetal bovine serum, 5% horse serum and 2 mM glutamine. Sema3A collapse assays For Sema3A collapse experiments, 450 ng ml −1 Sema3A (R&D Systems) or vehicle (phosphate-buffer saline, PBS plus 0.1% BSA) was only added to the axonal compartment. The concentration of Sema3A used was empirically determined to cause the maximal degree of collapse within 60 min. Drugs were applied to the axonal compartment concurrent with Sema3A treatment. The drugs were as follows: cycloheximide (1 μM, Sigma), anisomycin (40 μM, Sigma), MG132 (5 μM, Sigma), LLnL (50 μM, Sigma), lactacystin (10 μM, Sigma) and Y-27632 (10 μM, Calbiochem). Phase-contrast images of the same growth cones were taken before Sema3A application and 60 min after Sema3A or vehicle treatment. Only axons without varicosities or blebbing and whose growth cones remained healthy for the duration of the experiment were evaluated. Growth cones from axons that had bifurcated or growth cones that were contacting neighbouring axons were not analysed. Only growth cones that were not collapsed at the beginning of the experiment were analysed. A growth cone was considered collapsed if it had less than three filopodia, each shorter than 10 μm 5 . Because of the lower complexity of hippocampal growth cones, a growth cone was considered collapsed if it had less than two filopodia, each shorter than 5 μm. Washout between two sequential Sema3A collapse assays was achieved by rinsing the axonal compartment three times with Neurobasal and then applying complete medium supplemented with the experimental treatment to the axonal compartment only. The volume of media in the axonal compartment was kept 50 μl lower than in the cell body compartment to avoid the possibility of any axonal treatment spreading to the cell body compartment. Growth cones were considered morphologically recovered when they had more than three filopodia, each longer than 10 μm. Cycloheximide or anisomycin treatment prevented growth cone collapse when growth cones were pre-incubated with the drugs for 30 min or when the drugs were applied together with Sema3A. NGF outgrowth assays For NGF outgrowth assays, neurons were grown for 3DIV in growth media (50 ng ml −1 NGF) and then the media were exchanged to complete media containing 1 ng ml −1 of NGF in both the cell body and the axonal compartments for 16 h. For the assay, phase-contrast images of the same optical fields were taken before and 60 min after application of 0 or 50 ng ml −1 NGF. We empirically determined the minimum concentration of NGF that caused maximal axon outgrowth over 60 min. This concentration is consistent with that used in previous studies of NGF-induced axon outgrowth and protein synthesis in this neuronal culture system [7] . Only axons that remained healthy throughout the experiment and that did not bifurcate or fuse with nearby axons were analysed. The proteasome inhibitors LLnL (50 μM), lactacystin (10 μM) and MG132 (5 μM) were applied 30 min before exposure of axons to NGF. Image acquisition Images for collapse and outgrowth assays were acquired with a Nikon Ti2000 inverted microscope equipped with a BioPrecision2 motorized stage (Ludl Electronic Products) and a CoolSnap HQ digital CCD camera (Photometrics). All devices were controlled by NIS-Elements software (Nikon). A custom-made chamber for environmental control was used to maintain the cells at 37 °C and 5% CO 2 during image acquisition. The XYZ coordinates for each imaged optical field were recorded with NIS-Elements to allow fast re-loading of the same position after the 60-min incubation, keeping acquisition time to a very small fraction of the duration of the experiment (up to 5 min). Distal axons were imaged with a 10 × objective for outgrowth assays and with a 20 × objective for collapse assays. Immunostaining DRG neurons were rinsed with PBS, pH 7.4 and fixed with 4% paraformaldehyde in cytoskeletal buffer (60 mM PIPES, 27 mM HEPES, 10 mM EGTA and 4 mM MgSO 4 ) for 30 min at room temperature. After fixation, cells were permeabilized for 10 min with PBS/0.5% Triton X-100, cross-fixed for 5 min in 4% PFA in PBS, washed twice in PBS/0.1% Triton X-100 (PBST), blocked for 30 min in blocking buffer (PBST with 2% BSA), and labelled with primary antibodies in blocking buffer at 4 °C overnight. Coverslips were then washed three times with PBST and incubated with Alexa Fluor-conjugated secondary antibodies in blocking buffer for 1 h at room temperature. After incubation with secondary antibodies, coverslips were washed three times with PBST, rinsed with water and mounted on a glass microscope slide (VWR) with ProLong Gold with or without DAPI (Invitrogen). When staining for F-actin, cells were incubated with 488- or 568-Phalloidin (Invitrogen) in blocking buffer for 30 min at room temperature after secondary antibody incubation. Coverslips were then rinsed with PBST and mounted as described above. The following primary antibodies were used: K48-Ubiquitin (1:500, Millipore 05–1307), K63-Ubiquitin (1:250, Millipore 05–1308), Smurf1 (1:250, Abgent AP2104a), GAP43 (1:1,000, Millipore AB5220), tau-1 (1:500, Millipore MAB3420), RhoA (1:500, Santa Cruz Biotechnology sc-418), green fluorescent protein (GFP; 1:1,000, Abcam ab13970), 20S proteasome (1:250, Genetex GTX113530). Alexa Fluor-conjugated secondary antibodies (Invitrogen) were used at 1:1,000. Immunofluorescence images were collected using a Nikon Ti2000 inverted microscope with a CoolSnap CCD camera (Photometrics). Optimal exposure times were empirically determined for cell bodies or growth cones and for each antibody and kept constant and below grey scale saturation. Image acquisition was kept within the linear range of the camera by maintaining maximum fluorescence signals below 50% saturation of the photodetector CCD chip. Images were acquired as stacks (Z-step size=0.3 μm) using a × 60 Plan Apochromat oil immersion objective (numerical aperture 1.4). Stacks were then deconvolved with a 3D blind PSF algorithm (10 iterations) using AutoDeblur X software (AutoQuant). Post-acquisition image analysis and processing were performed with NIS-Elements (Nikon) and ImageJ (NIH) software. Briefly, deconvolved stacks were background subtracted using the mean pixel value of a non-cell region on each image with the statistical correction function in NIS-Elements. Then, regions of interest were selected using the counterstain channel, and fluorescence intensity per volume was measured for each of the fluorescent channels. Maximum intensity projections of the deconvolved stacks were generated and 16-bit images were converted to 8-bit copies solely for the purpose of figure assembly. Fluorescent time-lapse imaging DRG neurons for time-lapse experiments were cultured in medium without phenol red. Images for time-lapse experiments were acquired on a motorized Nikon TE2000 inverted microscope equipped with a custom chamber for environmental control that maintained the cells at 37 °C and 5% CO 2 for the duration of the experiment. Time-lapse images were acquired using a × 100 Plan Apochromat oil immersion objective (numerical aperture 1.4) and collected with a digital CCD camera (CoolSnap HQ2, Photometrics) using a 4 × 4 binning. Frames were collected every 400 ms and assembled after performing a background subtraction on each image. Generation and transduction of lentiviral constructs Replication-deficient lentiviruses were prepared using a third-generation lentiviral system [50] . Briefly, three helper plasmids (pLP1, pLP2, pVSV-G) and the vector containing the gene of interest with cis -acting sequences for proper packaging were used to generate pseudovirions. A subconfluent culture of HEK293T cells was transfected using the CalPhos Mammalian Transfection Kit (Clontech). The pseudoviral particles were purified and concentrated from the supernatant collected 24 and 48 h after transfection by ultracentrifugation at 22,000 r.p.m. ( ∼ 90,000 × g ) in a Beckman Coulter Centrifuge using a SW28.1 swinging-bucket rotor for 2 h. Viral pellets were resuspended in PBS containing 1% BSA, aliquoted and stored at −80 °C. The titre of each virus was determined using HEK293T cells. The overexpression constructs only included the coding sequence of the protein of interest. For infection of DRG neurons, pseudoviral particles were added to the culture 1 h after plating of the neurons, to allow neuronal cells to attach before transduction. Knockdown using shRNAs shRNAs were designed using iRNAi software (Mekentosj Inc.) to meet the following criteria: 19 nucleotides in length, 45–55% G/C content, higher free energy in the 3′ antisense region compared with the 5′ antisense region. To avoid off-target effects, a BLAST (NIH) homology search was performed on each candidate shRNA sequence. A minimum of four shRNAs were designed for each protein to be knocked down. shRNAs were cloned into the lentiviral plasmid to be expressed from an H1 promoter. The lentiviral plasmid also expressed GFP, and GFP expression was used to determine if a cell was infected. Pseudovirions were produced as described above. The efficacy of each shRNA was assessed by western blotting of endogenous protein from dissociated DRG cells transduced upon plating and cultured for 5 days to allow time for effective knockdown. The two shRNAs with the highest knockdown efficiency were selected for further experiments. The shRNA cassettes used to knock down rat Smurf1 mRNA (GenBank accession number NM_001109598 ) were: sh1 5′-GATCTCCGGTGGGAACTGCAGGTTTGTTCAAGAGACAAACCTGCAGTTCCCACCTTTTTAT-3′ and sh2 5′-GATCTCCACGGGGGCTTCACAGTTCCTTCAAGAGAGGAACTGTGAAGCCCCCGTTTTTTAT-3′. The non-targeting shLacZ cassette was 5′-GATCCCCGACTACACAAATCAGCGATTTCAAGAGAATCGCTGATTTGTGTAGTCTTTTTAT-3′. Western blotting Cells were lysed in RIPA buffer and proteins were resolved by 4–12% SDS–polyacrylamide gel electrophoresis (SDS–PAGE), electrotransferred to Immobilon-P polyvinylidene difluoride membranes (Millipore), blocked with 5% (w/v) nonfat milk, probed with the indicated primary antibodies, followed by incubation with HRP-conjugated secondary antibodies and detected by chemiluminescence. To assess knockdown of endogenous proteins by shRNAs, 300,000 dissociated DRG neurons were used and immunoreactivity was visualized using a digital imaging system (ChemiDoc MP, Bio-Rad). Protein quantification was performed using ImageLab (Bio-Rad) and ImageJ (NIH) software. The primary antibodies used in this study were as follows: Smurf1 (1:500, Sigma S341–353), β-actin (1:1,000, Genscript A00702), RhoA (1:1,000, Santa Cruz sc-179), Flag (1:1,000, Sigma F1804). HRP-conjugated secondary antibodies were used at 1:1,000–1:2,000. Where portions of gels are included in the main paper, uncropped scans are provided in the Supplementary Information . For pulldown experiments and immunoprecipitation, cells were lysed in lysis buffer (50 mM Tris-HCl (pH 7.4), 150 mM NaCl, 10% glycerol, 1% Triton X-100, 0.1% SDS) with protease inhibitor cocktail without EDTA. Pulldown experiments were performed with the Ni-NTA purification system or Dynabeads magnetic beads (Invitrogen) according to the manufacturer’s instructions. For RhoA immunoprecipitation, lysates were incubated with anti-RhoA mouse monoclonal antibody (Santa Cruz Biotechnology) for 3 h at 4 °C with rotation and then lysate-antibody solutions were incubated with magnetic beads for 3 h at 4 °C with rotation. Beads were separated using a magnet and washed four times before addition of SDS–PAGE sample buffer followed by boiling for 10 min. The recovered supernatant was separated on a 4–12% SDS–PAGE and transferred to a polyvinylidene difluoride membrane for western blotting. Spinal cord electroporation Electroporation of spinal cord explants was performed as previously described [7] , with minor modifications. Vertebral columns of CD-1 mouse E10.5 embryos were isolated in L15 medium and incubated with orbital shaking in 1 mg ml −1 dispase (Invitrogen) for 30 min at room temperature to dissociate spinal cords from the surrounding tissue. Open book explants were oriented with their dorsal side closest to the anode to preferentially target cell bodies in the dorsal root entry zone. To efficiently visualize electroporated axons, we used a construct in which enhanced green fluorescent protein (EGFP) expression was driven from a compound CAG promoter containing the chicken β-actin promoter, the minimum CMV enhancer and a large synthetic intron (a gift from Fred Gage’s laboratory). EGFP was co-electroporated with a construct expressing the non-degradable RhoA K6/7/51R mutant or the catalytically inactive Smurf1 C699A mutant. A total of 10 μg of DNA (1:1 GFP plasmid/mutant construct in case of co-electroporation) was electroporated with needle-style electrodes (BTX-Harvard Apparatus) using a square wave protocol (5 pulses of 50 ms, 20 V, 1 s interval). After electroporation, the spinal cord explants were embedded in 500 μl of collagen matrix (450 μl rat tail collagen (BD Biosciences), 55 μl 10 × DMEM, 45 μl sodium bicarbonate) and incubated for 30 min at 37 °C for solidification. After solidification of collagen, explants were cultured in Neurobasal supplemented with 1 × B27, 100 IU ml −1 penicillin, 100 mg ml −1 streptomycin and 2 mM glutamine. Two or three days after culturing, electroporated explants were removed from the collagen by incubation in collagenase type I (1 mg ml −1 , Affymetrix) for 30 min at 37 °C, fixed in 4% PFA in PBS for 40 min and mounted in ProLong Gold mounting medium (Invitrogen). Stacks of images were acquired using a Zeiss LSM 510 confocal microscope and processed with LSM 5 Image Examiner (Zeiss). Statistical analysis One-way analysis of variance with post-tests was used for the comparison of three or more groups, whereas unpaired, two-tailed Student’s t -test was used for the comparison of two groups. Error bars represent the standard error of the mean from a minimum of three independent experiments unless otherwise indicated. How to cite this article: Deglincerti, A. et al . Coupled local translation and degradation regulate growth cone collapse. Nat. Commun . 6:6888 doi: 10.1038/ncomms7888 (2015).